High-performance Raman quantum memory with optimal control in room temperature atoms 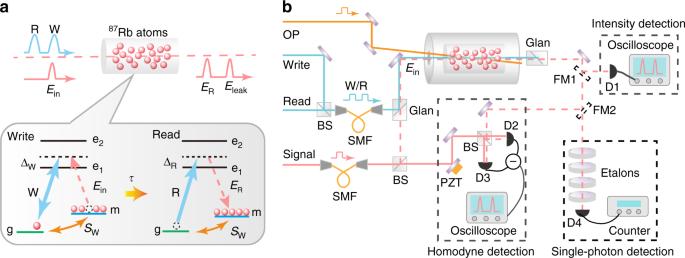Fig. 1 Raman memory.aSchematic, atomic energy levels and frequencies of the optical fields. |g,m〉: hyperfine levels |52S1/2,F= 1, 2〉; |e1〉 and |e2〉: excited states |52P1/2,F= 2〉 and |52P3/2〉. W write field,Eininput signal,Eleakleaked signal,SWcollective atomic spin wave, R read field,ERretrieved signal.bExperimental setup. The polarizations of the weak signal beams,EinandER, are perpendicular to the strong driving beams, W and R. The signals can be detected by homodyne detection. OP optical pumping laser, SMF single-mode fiber, BS beam splitter, PZT piezoelectric transducer. D1 photo-detector, D2 and D3 photo-diode, D4 single-photon detector, FM1 and FM2 flip mirror. The flip mirrors FM1,2 allow alternative selection of detections via intensity, homodyne, and single photon. Intensity detection is chosen to calibrate the memory efficiency by flipping FM1 up, homodyne detection combining with tomography reconstruction to determine the memory fidelity by flipping FM1 down and FM2 up, and single-photon detection to measure and analyze the excess noise in storage process by flipping FM1,2 both down Quantum memories are essential for quantum information processing. Techniques have been developed for quantum memory based on atomic ensembles. The atomic memories through optical resonance usually suffer from the narrow-band limitation. The far off-resonant Raman process is a promising candidate for atomic memories due to broad bandwidths and high speeds. However, to date, the low memory efficiency remains an unsolved bottleneck. Here, we demonstrate a high-performance atomic Raman memory in 87 Rb vapour with the development of an optimal control technique. A memory efficiency of above 82.0% for 6 ns~20 ns optical pulses is achieved. In particular, an unconditional fidelity of up to 98.0%, significantly exceeding the no-cloning limit, is obtained with the tomography reconstruction for a single-photon level coherent input. Our work marks an important advance of atomic memory towards practical applications in quantum information processing. Quantum memory is a necessary component for quantum communications and quantum computing. A practical quantum memory should be efficient, low-noise, broadband, and as simple as possible to operate [1] , [2] , [3] , [4] , [5] , [6] . Using several approaches, including electromagnetically induced transparency (EIT), gradient echo memory (GEM), the off-resonant Faraday effect, and far off-resonant Raman memory, optical memory has been demonstrated in cold atomic ensembles [2] , [7] , [8] , [9] , atomic vapors [10] , [11] , [12] , [13] , [14] , and solids [15] , [16] , [17] , [18] , [19] . Hsiao et al. [20] reported a 92.0% memory efficiency for a coherent light pulse in a cold atomic ensemble using EIT. Hosseini et al. [21] used GEM to realize a 78% memory efficiency for weak coherent states with 98% fidelity. Polzik’s group [12] demonstrated a quantum memory with a fidelity of 70% based on the off-resonant Faraday effect. These examples [12] , [20] , [21] successfully demonstrated the capability to store optical states with high efficiency and/or fidelity exceeding the classical limit [22] , [23] , [24] and sub-megahertz bandwidths. However, the bandwidth is important for the practical application of quantum memory [25] . Quantum sources with bandwidth at the GHz level have been used in long-distance quantum communication [26] , [27] and quantum computers [28] . Unlike these protocols, far-off-resonant atomic Raman memory can store short-time pulses corresponding to high bandwidths and can operate at high speeds. In addition, the far-off-resonance characteristic makes the atomic Raman memory [10] , [29] , [30] robust against inhomogeneities in the ensemble and facilitates controlling the frequency of the output state. All of these properties indicate that atomic Raman memory has great potential in practical quantum information processing. The first experimental realization of an atomic Raman memory was demonstrated [29] in 2010. This indeed represented significant progress in the field of Raman memory, but the limitations with low efficiency (<30%) and significant noise from the spontaneous four-wave mixing (FWM) process persist. Recently, Raman memory using photonic polarized entanglement [30] was reported in a cold atomic ensemble with a fidelity of 86.9 ± 3.0%, but still an efficiency of only 20.9 ± 7.7%. An efficiency exceeding 50% and a fidelity exceeding 2/3 are necessary to store and retrieve an optical state within the no-cloning regime without post-selection [22] , [23] , [24] , [31] . Therefore, so far, low efficiency has appeared to exclude the broadband Raman memory as an unconditional quantum memory. In this paper, we present an optimal control technique where the atomic vapor is performed a real-time optimal response on an input signal pulse. With a 87 Rb atomic vapor in paraffin-coated cell at T = 78.5 °C, we achieve a Raman quantum memory on a coherent input of 6–20 ns duration with above 82.0% memory efficiency, and more importantly, with 98% unconditional fidelity at single photon level ( n ≈ 1). Experimental setup The experimental setup and atomic levels are depicted in Fig. 1 . The 87 Rb atomic vapor in the paraffin-coated glass cell is the core component of the current Raman memory. The atomic cell is 10.0 cm long, has a diameter of 1.0 cm, and is heated to 78.5 °C. Our Raman memory starts with a large ensemble of atoms that were initially prepared in the | m 〉 = |5 2 S 1/2 , F = 2〉 state by a 44-μs-long optical pumping pulse (OP). Then, the input signal pulse E in is stored as atomic spin excitation S W induced by the strong off-resonant write pulse (W) with the Rabi frequency Ω W ( t ) and detuning Δ W . After a certain delay τ , the atomic excitation can be retrieved into optical state E R by the strong off-resonant read pulse (R) with the Rabi frequency Ω R ( t ) and detuning Δ R . The waists of the laser beams (W, R, and E in ) are all 600 μm. The two strong driving beams, W and R, can be generated by the same or different semiconductor lasers (Toptica, DLPro + Boosta) and are coupled into the same single-mode fiber. Their intensities and temporal shapes are controlled by acousto-optic modulators (AOMs). The input E in signal comes from another semiconductor laser (Toptica, DLPro) phase-locked on the W laser. The temporal shape is controlled by a Pockels cell (Conoptics, Model No. 360-80). The shortest pulse duration of the Pockels cell is 6 ns. The W and E in fields are two-photon resonant and spatially overlapped after passing through a Glan polarizer with 94% spatial visibility in the atomic vapor. The output signals can be separated from the strong driving pulses by another Glan polarizer with an extinction ratio of 40 dB, and detected, respectively, by intensity detection to calibrate the memory efficiency, by homodyne detection combining with tomography reconstruction to determine the memory fidelity, and by single-photon detection to analyze the excess noise in storage process. The total optical transmittance including the atomic cell and all optical elements in homodyne detection is about 89%. The four etalons with 33% transmission can filter the leaked driving photons at 115 dB. Fig. 1 Raman memory. a Schematic, atomic energy levels and frequencies of the optical fields. | g , m 〉: hyperfine levels |5 2 S 1/2 , F = 1, 2〉; | e 1 〉 and | e 2 〉: excited states |5 2 P 1/2 , F = 2〉 and |5 2 P 3/2 〉. W write field, E in input signal, E leak leaked signal, S W collective atomic spin wave, R read field, E R retrieved signal. b Experimental setup. The polarizations of the weak signal beams, E in and E R , are perpendicular to the strong driving beams, W and R. The signals can be detected by homodyne detection. OP optical pumping laser, SMF single-mode fiber, BS beam splitter, PZT piezoelectric transducer. D1 photo-detector, D2 and D3 photo-diode, D4 single-photon detector, FM1 and FM2 flip mirror. The flip mirrors FM1,2 allow alternative selection of detections via intensity, homodyne, and single photon. Intensity detection is chosen to calibrate the memory efficiency by flipping FM1 up, homodyne detection combining with tomography reconstruction to determine the memory fidelity by flipping FM1 down and FM2 up, and single-photon detection to measure and analyze the excess noise in storage process by flipping FM1,2 both down Full size image Efficiency The Raman write process is a type of coherent absorption induced by a strong write pulse. As shown in Fig. 2a , when the write pulse is switched off, owing to the far-off-resonant frequency, almost 100% of the E in pulse passes through the atomic vapor. Below, we use the total energy of such an E in pulse to normalize the write and retrieve efficiencies. When the write pulse is turned on, part of the energy of the E in pulse is converted coherently as the atomic spin wave S W ( z ) near the two-photon resonance frequency. The rest of the E in energy passes through the atoms as E leak , as shown in Fig. 1a . The full width at half maximum (FWHM) of the absorption spectrum is approximately 100 MHz, as shown in Fig. 2a . Fig. 2 Efficient Raman memory. a Absorption rate of the weak input-signal pulse as a function of the Raman detuning frequency. Δ W is fixed at 3.0 GHz. The input signal pulse is 10 ns long. b Theoretical efficiency as a function of the energy of the strong control pulse. The input optical pulse is a 10 ns near-square pulse. All optical fields detune 3.0 GHz from atomic transition and the optical depth d = 1100 (see Methods section for details). In the write process, the efficiency is always much smaller than 1.0 when using a non-optimal write pulse (10 ns Gaussian shape), but it can approach 1.0 with the optimal write pulse when the write pulse is larger than 1.5 nJ. In the read process, the curves with Gaussian and square read pulses coincide with each other. The retrieval efficiency is waveform-independent and increases with the energy of the read pulse until approaching 1.0. c Temporal modes of the strong driving (blue, experimental shape of write pulse \(W_{{\mathrm{exp}}}^{{\mathrm{opt}}}\) , read pulse R ; dashed purple, theoretical shape of optimal write pulse \(W_{{\mathrm{theory}}}^{{\mathrm{opt}}}\) ), input signal (black, E in ), leaked signal (orange, E leak ), and output signal (red, E R ) pulses. d Waveform of the leaked signal with the \(W_{{\mathrm{exp}}}^{{\mathrm{opt}}}(t)\) (orange circle) and \(W_{{\mathrm{exp}}}^{{\mathrm{opt}}}(t + 1ns)\) (gray square) write pulse. The lines are the corresponding theoretical fits. e Storage efficiency ( η W ) and retrieval efficiency ( η R ) as function of the energy of the driving pulse (W and R) with the shape of \(W_{{\mathrm{exp}}}^{{\mathrm{opt}}}\) and R as shown in ( c ). Square represents experimental data and solid line is theoretical fitting. The error bars correspond to one standard deviation caused by the statistical uncertainty of measurement. f The write-in efficiency as a function of the width of the E in pulse Full size image According to the theoretical analysis in ref. [32] , the spatial-distributed atomic spin wave in a far-off-resonant Raman write process is given by 
    S_W(z) = ∫_0^t_W q(z,t)E_in(t)dt,
 (1) where \(q(z,t) = i\frac{{\sqrt d }}{{{\mathrm{\Delta }}_{\mathrm{W}}}}{\mathrm{\Omega }}_{\mathrm{W}}^ \ast (t)e^{i\frac{{dz + h(t,t_{\mathrm{W}})}}{{{\mathrm{\Delta }}_{\mathrm{W}}}}}J_0\left( {\frac{{2\sqrt {h(t,t_{\mathrm{W}})dz} }}{{{\mathrm{\Delta }}_{\mathrm{W}}}}} \right)\) , t W is the duration of the write process, d is the optical depth of atomic ensemble, and \(h(t,t_{\mathrm{W}}) = {\int}_t^{t_{\mathrm{W}}} \left| {{\mathrm{\Omega }}_{\mathrm{W}}(t^\prime )} \right|^2dt^\prime\) with t ′ is the integration variable from t t o t W in the co-moving frame. Eq. ( 1 ) is an iterative function that is determined by the matching between the temporal shapes of the input E in ( t ) and the write pulse Ω W ( t ) [32] , [33] , [34] . Therefore, to achieve efficient conversion, it is crucial to perform real-time control on Ω W ( t ) or E in ( t ) to make the atoms coherently absorb as much energy E in ( t ) as possible. The optimal control of E in ( t ) has been used to achieve efficient memory in an EIT-based process [20] , where the shape of the input signal E in ( t ) was adjusted according to atomic memory system. Here, we prefer the dynamical control Ω W ( t ) because a quantum memory system should have the ability to store and preserve quantum information of an input optical signal with an arbitrary pulse shape. To obtain the optimal Ω W ( t ), denoted \(\Omega _{\mathrm{W}}^{{\mathrm{opt}}}(t)\) , we first use the iterative methods mentioned in ref. [32] to calculate the optimal spin wave, corresponding to the minimum E leak . Then, the optimal spin wave establishes a one-to-one correspondence between E in ( t ) and \(\Omega _{\mathrm{W}}^{{\mathrm{opt}}}(t)\) via Eq. ( 1 ). Thus, for any given shape of E in ( t ), \(\Omega _{\mathrm{W}}^{{\mathrm{opt}}}(t)\) can be obtained from Eq. ( 1 ) via the optimal spin wave. Moreover, the corresponding optimal efficiency \(\eta _{\mathrm{W}}^{{\mathrm{opt}}}\) depends only on the optical d epth d and the total energy of the write pulse. 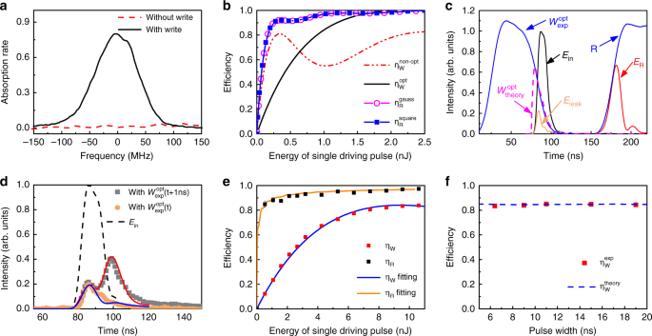Fig. 2 Efficient Raman memory.aAbsorption rate of the weak input-signal pulse as a function of the Raman detuning frequency. ΔWis fixed at 3.0 GHz. The input signal pulse is 10 ns long.bTheoretical efficiency as a function of the energy of the strong control pulse. The input optical pulse is a 10 ns near-square pulse. All optical fields detune 3.0 GHz from atomic transition and the optical depthd= 1100 (see Methods section for details). In the write process, the efficiency is always much smaller than 1.0 when using a non-optimal write pulse (10 ns Gaussian shape), but it can approach 1.0 with the optimal write pulse when the write pulse is larger than 1.5 nJ. In the read process, the curves with Gaussian and square read pulses coincide with each other. The retrieval efficiency is waveform-independent and increases with the energy of the read pulse until approaching 1.0.cTemporal modes of the strong driving (blue, experimental shape of write pulse\(W_{{\mathrm{exp}}}^{{\mathrm{opt}}}\), read pulseR; dashed purple, theoretical shape of optimal write pulse\(W_{{\mathrm{theory}}}^{{\mathrm{opt}}}\)), input signal (black,Ein), leaked signal (orange,Eleak), and output signal (red,ER) pulses.dWaveform of the leaked signal with the\(W_{{\mathrm{exp}}}^{{\mathrm{opt}}}(t)\)(orange circle) and\(W_{{\mathrm{exp}}}^{{\mathrm{opt}}}(t + 1ns)\)(gray square) write pulse. The lines are the corresponding theoretical fits.eStorage efficiency (ηW) and retrieval efficiency (ηR) as function of the energy of the driving pulse (W and R) with the shape of\(W_{{\mathrm{exp}}}^{{\mathrm{opt}}}\)and R as shown in (c). Square represents experimental data and solid line is theoretical fitting. The error bars correspond to one standard deviation caused by the statistical uncertainty of measurement.fThe write-in efficiency as a function of the width of theEinpulse 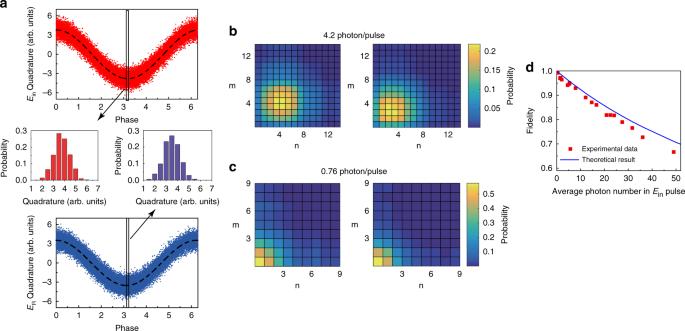Fig. 3 Fidelity of the Raman memory.aQuadrature amplitudes of the input and output signal pulses at an average of 7.9 photons/pulse. Insets are the probability distributions of theEinandERquadrature values at the indicated phase. The density matrices of the input and output signal pulses at 4.2 (b) and 0.76 (c) photons/pulse on average.dFidelity as a function of the number of photons contained in the input signal pulse. The red squares show the experimental data, and the black line shows the theoretical result. The error bars correspond to one standard deviation caused by the measurement noise Figure 2b shows the theoretical efficiencies as the function of the energy of the strong driven pulses. Using a 10 ns near-square pulse as the input E in , the write efficiency with \(\Omega _{\mathrm{W}}^{{\mathrm{opt}}}(t)\) is approximately equal to 1 when the energy of a write pulse with 10 ns duration is larger than 1.5 nJ, while the maximum write-in efficiency with a non-optimized Ω W ( t ) (a 10 ns Gaussian-shaped Ω W ( t ) is used in Fig. 2 ) is much smaller than one. In the read process (see Fig. 1 ), the spin wave S W ( z ) is retrieved back to the optical field E R ( t ) by the read pulse Ω R ( t ). Unlike η W , the retrieval efficiency η R is independent of the temporal waveform [32] , and a read pulse whose duration is 10 ns with strong power but without temporal optimization is sufficient for η R ~ 1. This can be seen in Fig. 2b . η R increases with the total energy of the read pulse, whether Gaussian or square-shaped until η R ~ 1. Thus, with the above optimal control on Ω W ( t ), the total efficiency of the Raman memory process is η T = η W × η R ~ 1 in principle. Here, we experimentally demonstrate a break of the efficiency in Raman memory with dynamic control over the temporal shape of the write pulse. In the experiment, the given E in pulse is mapped in a forward-retrieval configuration. We derive \(\Omega _{\mathrm{W}}^{{\mathrm{opt}}}(t)\) using the iteration-based optimization strategy based on the given short E in ( t ) pulse and experimentally control the temporal profile of the write pulse by using an intensity modulator (here, an AOM). The theoretical shape of optimal write pulse \(W_{{\mathrm{theory}}}^{{\mathrm{opt}}}\) and the experimentally-optimized shape \(W_{{\mathrm{exp}}}^{{\mathrm{opt}}}\) are given in Fig. 2c . The experimental shape is much longer than the theoretical one before the E in pulse is turned on due to the limitation of the bandwidth of our intensity modulator, but two curves match well within the E in duration effectively guaranteed high write-in efficiency. Furthermore, to show the definite improvement of optimization control, two write pulses are given, the optimal \(W_{{\mathrm{exp}}}^{{\mathrm{opt}}}(t)\) and an optimal write pulse delayed by 1.0 ns, \(W_{{\mathrm{exp}}}^{{\mathrm{opt}}}\left( {t + 1\,{\mathrm{ns}}} \right)\) . The corresponding leaked optical pulses and the theoretical fits are shown in Fig. 2d . The leaked energy for the sub-optimal curve is twice that for the optimal one. Through the optimal control, the leaked energy of the input signal is greatly reduced. The storage efficiency η W , calculated by \((\overline N _{E_{{\mathrm{in}}}} - \overline N _{E_{{\mathrm{leak}}}})/\overline N _{E_{{\mathrm{in}}}}\) , reaches ~84% when the atomic temperature T is 78.5 °C and the power of the write pulse is 10.6 nJ (Fig. 2e ). Such high a write-in efficiency can be achieved when the signal duration changes from 6 to 20 ns, and η W always remains above 83.5% by optimal control, as shown in Fig. 2f . The retrieval efficiency η R , calculated by \(\left( {\overline N _{E_{\mathrm{R}}}/(\overline N _{E_{{\mathrm{in}}}} - \overline N _{E_{{\mathrm{leak}}}})} \right)\) , can reach 98.5% when the read laser is 10.6 nJ, with 3.0 GHz frequency detuning (Fig. 2e ). Here, E in , E leak , and E R pulses are all measured through the intensity detection as shown in Fig. 1b . The optical paths for these pulses are arranged in the way that they are subject to the same optical losses. This allows the storage efficiency to be calibrated to characterize the atomic memory process alone. The total memory efficiency, η T = η W × η R , is above 82.0% when the input signal pulse contains an average number of photons ranging from 0.4 to 10 4 ; thus, this Raman memory is a good linear absorber. The 82.0% memory efficiency is the best performance reported to date for Raman-based memory and far exceeds the no-cloning limit. In principle, η T = η W × η R ~ 1. With η R = 98.5%, further improvement of η T mainly depends on η W , which could be improved by better experimental conditions. According to our theoretical analysis, larger atomic optical depth through increasing the atomic temperature or lengthening the cell could lead to about 3% improvement. Better temporal-mode control on the W pulse may bring about 6% increase. Improving the spatial-mode match between the E in and W beams can contribute about 5%. Fidelity Fidelity is the ultimate performance criterion for quantum memory and reflects the maintenance of the quantum characteristics of the optical signal during the memory process. At the few-photon level, fidelity is readily degraded by excess noise and is mainly caused by the FWM process [10] and spontaneous emission. Spontaneous noise comes from the spontaneous Raman scattering between the strong write pulse and the atoms populating the | g 〉 = |5 2 S 1/2 , F = 1〉 state. Having fewer | g 〉 atoms helps suppress the spontaneous excess noise. In our paraffin-coated cell, more than 98% of the atoms populate the | m 〉 state. The spontaneous emission noise intensity is measured by determining the photon number using the single-photon detection as shown in Fig. 1b when the E in pulse is turned off. On average, the spontaneous noise is approximately 0.02 photons per memory process at the end of the atomic cell for two strong driving pulses with a power of 10.6 nJ at a detuning frequency of 3.0 GHz. The FWM excess noise is mainly attributed to anti-Stokes ( AS FWM , with same frequency of E R ) and Stokes ( S FWM ) photons with the same intensity. We can deduce the proportion of AS FWM in retrieved E R pulse by measuring the intensity of S FWM using single-photon detection. Our results show that the AS FWM noise is less than 10% in E R . Such low excess noise effectively guarantees the fidelity of the quantum memory process. To achieve the fidelity performance of the current Raman quantum memory, we measure the fidelity using the equation \(F = \left| {Tr\left( {\sqrt {\sqrt {\rho _{{\mathrm{in}}}} \rho _{{\mathrm{out}}}\sqrt {\rho _{{\mathrm{in}}}} } } \right)} \right|^2\) [35] , where ρ in and ρ out are the reconstructed density matrices of E in and E R , respectively. We record the quadrature amplitudes of the E in and E R signals using homodyne measurement, and we then reconstruct the density matrices by tomographic reconstruction [36] . The setup used for homodyne detection is shown in Fig. 1b . To stabilize the phase difference between the E in and E R pulses and simplify the homodyne setup, the write and read pulses are generated by the same laser and are controlled using one intensity modulator. In the measurement, the two weak signals, E in and E R , are both short pulses. Matching the temporal modes of short pulses is difficult. Therefore, we use a strong continuous laser beam with the same frequency as the signal pulses E in and E R as the local oscillator for homodyne detection (the detailed strategy can be found in refs. [36] , [37] ). We recorded 10 5 sets of quadrature amplitudes of the E in and E R pulses while varying the phase of the local oscillator between 0 and 2 π by scanning the piezoelectric transducer, multiplying the quadrature amplitudes of each pulse by the temporal shapes of the corresponding signals, and finally, integrating the product over the signal pulse duration. The temporal shape functions of the E in and E R pulses are obtained by pointwise variance method. The integrated quadrature amplitude, which is normalized with the vacuum, as a function of the local oscillator phase is shown in Fig. 3a , where the mean number of photons contained in the E in pulse is 7.9. The phase of the retrieved E R signal pulse closely follows that of the input E in pulse. Insets in Fig. 3a are the probability distributions of amplitude quadratures of the E in and E R pulses showing good Gaussian distributions. Fig. 3 Fidelity of the Raman memory. a Quadrature amplitudes of the input and output signal pulses at an average of 7.9 photons/pulse. Insets are the probability distributions of the E in and E R quadrature values at the indicated phase. The density matrices of the input and output signal pulses at 4.2 ( b ) and 0.76 ( c ) photons/pulse on average. d Fidelity as a function of the number of photons contained in the input signal pulse. The red squares show the experimental data, and the black line shows the theoretical result. The error bars correspond to one standard deviation caused by the measurement noise Full size image The density matrix elements of the E in and E R pulses are obtained based on the quadrature-amplitude results using the maximum-likelihood reconstruction method [36] , [38] . Then on the basis of the diagonal density matrix elements, the photon distributions of the input and output pulses can be achieved to calculate the average photon numbers. The results are plotted in Fig. 3b, c , with the input pulses containing, on average, 4.2 and 0.76 photons, corresponding to unconditional fidelities of 0.915 and 0.98, respectively. The fidelities significantly exceed the no-cloning limit, indicating that the current Raman memory is a quantum-memory process and does not introduce significant excess noise during the memory process. As mentioned above, the current Raman memory is a good linear absorber and allows the storage and retrieval of coherent optical signals at the single-photon level for up to 10 4 photons with the same memory efficiency. Unlike the efficiency, the unconditional fidelity of the quantum memory of the coherent field is related to the average photon number contained in the input signal \(\left( {\overline N _{E_{{\mathrm{in}}}}} \right)\) and efficiency ( η T ) by \(F = 1/\left[ {1 + \overline N _{E_{{\mathrm{in}}}}(1 - \sqrt {\eta _{\mathrm{T}}} )^2} \right]\) [24] , which shows that if η T < 1, the fidelity will rapidly decrease with \(\overline N _{E_{{\mathrm{in}}}}\) owing to the worse overlap between ρ in and ρ out . In Fig. 3d , the fidelity is shown as a function of \(\overline N _{E_{{\mathrm{in}}}}\) with η T = 82.0%. The experimental F value is slightly smaller than the theoretical F value because of the excess noise in the experiment. F exceeds the no-cloning limit [22] , [23] , [24] at \(\overline N _{E_{{\mathrm{in}}}} \le 49\) in the current Raman memory process. Bandwidth and coherence time Far off-resonant Raman memory is a genuine broadband memory. The ability to store and retrieve broadband pulses was successfully demonstrated in ref. [29] , where a bandwidth larger than 1 GHz of the retrieved signal was obtained using a 300 ps and 4.8 nJ read pulse. In a practical Raman memory, the bandwidth is generated dynamically by the strong driving pulses. In Fig. 2 , the shortest E in pulse has a FWHM of 6 ns and a bandwidth of 170 MHz. The FWHM of the E R signal pulse which mainly depends on the rise time of the R pulse is 13 ns, corresponding to a bandwidth of 77 MHz. The bandwidth in the current memory is dozens or hundreds of times larger than the values reported based on the EIT [20] , Faraday [12] , and GEM [21] approaches, thus demonstrating the broadband memory ability of the current quantum memory scheme. In our experiment, the memory bandwidth is limited by the currently available intensity modulators (AOM and Pockels cell) and the corresponding electronics controllers (arbitrary wave generators) in our lab. The duration limit of the Pockels cell is 6 ns. As shown in Fig. 2f , the write-in efficiencies remain above 83.5% as the signal duration is larger than 6 ns. Shorter E in and E R pulses corresponding larger bandwidths need faster intensity modulators and electronics controllers. The decoherence time, which is another essential criterion for good quantum memory, is measured to be approximately 1.1 μs. The delay-bandwidth product at 50% memory efficiency, an appropriate figure of merit, is defined as the ratio of the memory time to the duration of the signal pulse and is 86 in this work. In the present atomic system, the decoherence time is mainly limited by the atomic diffusion out of the laser beam [39] . The delay-bandwidth product could be increased to ~10 3 by using a shorter signal pulse and an anti-relaxation-coated cell with the same diameter of the millimeter order as the laser beams. This can lead to a typical decoherence time of approximately several microseconds [40] . In summary, we have demonstrated a high-performance broadband quantum optical memory via pulse-optimized Raman memory in free space. The 82.0% memory efficiency is the highest value obtained to date for far-off-resonant Raman memory. The unconditional fidelity of 98% for an input pulse containing an average of approximately one photon significantly exceeds the classical limit. The 77 MHz bandwidth of the current memory is dozens or hundreds of times larger than the reported bandwidths for memories based on the EIT, Faraday, and GEM approaches. The delay-bandwidth product at 50% memory efficiency is 86. These attractive properties demonstrate that the Raman memory is a high-performance broadband quantum memory. Additionally, our memory is implemented in an atomic vapor system that can be easily operated and could become the core of a scalable platform for quantum information processing, long-distance quantum communication and quantum computation. Optical depth The formula of the optical depth is d = g 2 NL /( γc ) [32] , where g is the atom-field coupling constant, N is the number of atoms, L is the length of atomic ensemble, γ is the decay rate of the | e 1 〉, and c is the speed of light. The values of these parameters are: g = 6.79 × 10 4 s −1 and γ = 3.613 × 10 7 s −1 for 87 Rb D1 line, L = 10 cm, c = 3 × 10 8 m ⋅ s −1 . The number of atoms varies with the temperature of the vapor cell. According to fluorescence measurement in experiment [41] , N ~ 2.58 × 10 10 at the cell temperature of 78.5 °C.